Coordination of biradial-to-radial symmetry and tissue polarity by HD-ZIP II proteins 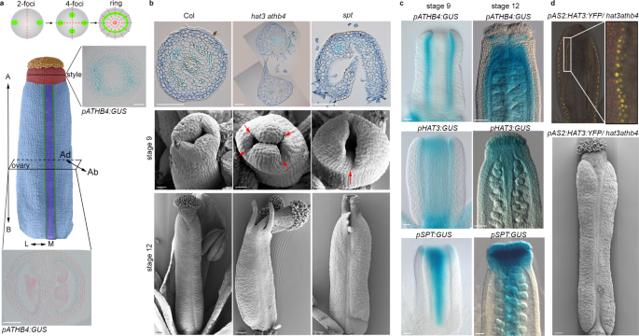Fig. 1: HD-ZIP II proteins HAT3 and ATHB4 coordinate adaxial/abaxial polarity axis during symmetry transition. aSchematic representation of symmetry transition in Arabidopsis wild-type gynoecium (Col-0); (top) schematic indicating the dynamic distribution of theDR5rev::GFPsignal in the outline of the gynoecium viewed from the top. Two-foci = bilateral symmetry—one plane of symmetry; four-foci = biradial symmetry—two planes of symmetry; ring = radial symmetry—≥3 planes of symmetry; (bottom) false-coloured scanning electronic micrograph (SEM) of wild type at stage 11. Stigma (orange), style (red), valves (light blue), valve margins (green), replum (violet), including GUS-stained cross-sections of thepATHB4:GUSreporter shown for radially symmetric style (top) and bilaterally symmetric ovary (bottom). Scale bars represent 50 µm. Double-headed arrows indicate the polarity axes: A apical, B basal, M medial, L lateral, Ab abaxial, Ad adaxial.bOptical images of Toluidine blue-stained cross-sections of stage-12 style (top panels; scale bars represent 100 μm) and SEM images (middle and bottom panels) of Col-0 (left),hat3 athb4(centre) andspt(right) at stage 9 (middle; scale bars represent 20 μm) and stage 12 (bottom; scale bars represent 100 μm). Red arrows indicate the different positions of the split style in the mutant backgrounds.cOptical images of GUS-stained gynoecia ofpATHB4:GUS(top),pHAT3:GUS(middle) andpSPT:GUS(bottom) lines at stage 9 (left) and stage 12 (right) of gynoecium development. Scale bars represent 20 µm (left, stage 9) and 50 µm (right, stage 12).b,cSimilar results were obtained from four independent experiments. Sections in (a,b) were made using samples from two of the four biological replicates in (b,c).dConfocal (top) and SEM (bottom) images ofpAS2:HAT3:YFP/hat3 athb4gynoecia at stage 9 (top) and stage 12 (bottom) of development. Scale bar represents 100 µm. Similar results were obtained from three independent experiments. Symmetry establishment is a critical process in the development of multicellular organs and requires careful coordination of polarity axes while cells actively divide within tissues. Formation of the apical style in the Arabidopsis gynoecium involves a bilateral-to-radial symmetry transition, a stepwise process underpinned by the dynamic distribution of the plant morphogen auxin. Here we show that SPATULA (SPT) and the HECATE (HEC) bHLH proteins mediate the final step in the style radialisation process and synergistically control the expression of adaxial-identity genes, HOMEOBOX ARABIDOPSIS THALIANA 3 ( HAT3 ) and ARABIDOPSIS THALIANA HOMEOBOX 4 ( ATHB4 ). 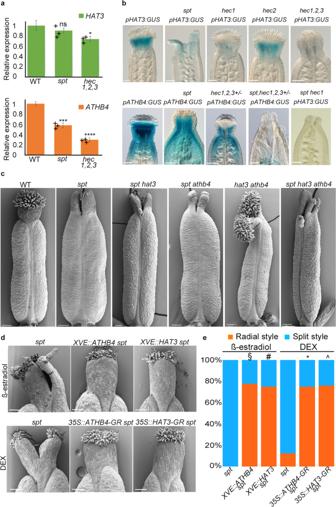Fig. 2: SPT/HEC synergistic control ofHAT3andATHB4expression and genetic analyses. aqRT-PCR ofHAT3andATHB4in Col-0,sptandhec1,2,3mutant inflorescences normalised againstUBIQUITIN10. The centre for the error bars represents mean, while error bars represent SD; *p< 0.05, ***p< 0.001, ****p< 0.0001, ns indicates no statistically significant difference (two-sided Student’sttest),n= 3 technical replicates. The panel displays similar results obtained from one of three biological replicates analysed, and up to six technical replicates for each gene and for each biological replicate were performed.bOptical images of stage-12 gynoecia showingpHAT3:GUS(top) andpATHB4:GUS(bottom) expression in Col-0,sptand combinations ofhec1,2,3andsptmutants, as depicted on individual panels.cSEM images of stage-12 gynoecia of Col-0,spt,spt hat3,spt athb4,hat3 athb4andspt hat3 athb4. Scale bars represent 100 µm.b,cSimilar results were obtained from three independent experiments.dSEM images of stage-13 styles ofATHB4(XVE::ATHB4and35S::ATHB4:GR) andHAT3(XVE::HAT3and35S::HAT3:GR) overexpression lines insptbackground, treated with either 20 µM β-estradiol (top) or 10 µM DEX (bottom). Scale bars represent 100 µm.eQuantification of the radial (orange bars) and split (blue bars) style phenotype ofHAT3andATHB4overexpression lines (XVE::HAT3,XVE::ATHB4,35S::HAT3:GRand35S::ATHB4:GR)insptbackground treated with mock, β-estradiol and DEX. Phenotypic classes were compared using contingency 2 × 2 tables followed by Pearson’sχ2test. Two-tailedPvalues are as follows:spt-12 XVE::ATHB4β-estradiol vsspt-12β-estradiolP< 0.00001 (§);spt-12 XVE::HAT3β-estradiol vsspt-12β-estradiolP< 0.00001 (#);spt-12 35S::ATHB4:GRDEX vsspt-12DEXP< 0.00001 (*);spt-12 35S::HAT3:GRDEX vsspt-12DEXP< 0.00001 (^).Pvalues < 0.01 were considered as extremely statistically significant. HAT3/ATHB4 module drives radialisation of the apical style by promoting basal-to-apical auxin flow and via a negative feedback mechanism that finetune auxin distribution through repression of SPT expression and cytokinin sensitivity. Thus, this work reveals the molecular basis of axes-coordination and hormonal cross-talk during the sequential steps of symmetry transition in the Arabidopsis style. A major challenge during organ morphogenesis includes the establishment of symmetries along the organ polarity axes (apical–basal, medio-lateral and dorso-ventral/abaxial–adaxial) [1] , [2] , [3] , [4] , [5] . We have previously shown that the female reproductive organ (gynoecium) of Arabidopsis thaliana provides an excellent model for symmetry studies during organogenesis [6] , [7] (Fig. 1a ). At early developmental stages, the ovary of the Arabidopsis gynoecium is bilaterally symmetric (one plane of symmetry) reflecting the congenital fusion of two carpels [8] , [9] (Fig. 1a ). Later, a transition in symmetry occurs, when the apical end becomes radially symmetric [6] (three or more planes of symmetry) (Fig. 1 ), thus forming the style. We have shown that the overall bilateral-to-radial symmetry transition observed at the organ level is guided by consecutive transitions in the distribution of the plant hormone auxin, which includes a biradial state [6] . Initially, auxin accumulates in two lateral foci (two-foci stage) at the apex of the gynoecium in accordance with the inherent bilateral symmetry at this stage [6] (Fig. 1a ). Subsequently, two new medial foci form (four-foci stage) establishing a biradially symmetric state of auxin distribution (two planes of symmetry at 90° to each other), before a continuous, ring-formed, auxin signalling maximum provides information for radial symmetry [6] (Fig. 1a ). The requirement for this precise spatio-temporal pattern of auxin dynamics is well-established and controls the axisymmetric growth and patterning of tissues along the apical–basal and medio-lateral axes [5] , [6] , [10] , [11] , during the developmental transitions of the gynoecium. It is, however, still unresolved how this dynamic auxin pattern is coordinated with the adaxial–abaxial polarity axis during the radialisation process, within the radially symmetric style. In this paper, we present experiments suggesting a two-step mechanism whereby stage-specific transcription factor complexes control the timely expression of polarity identity genes to coordinate hormone distribution and sensitivity. The proposed mechanism therefore provides a framework for the integration of gene regulatory and hormonal activities during organogenesis. Fig. 1: HD-ZIP II proteins HAT3 and ATHB4 coordinate adaxial/abaxial polarity axis during symmetry transition. a Schematic representation of symmetry transition in Arabidopsis wild-type gynoecium (Col-0); (top) schematic indicating the dynamic distribution of the DR5rev::GFP signal in the outline of the gynoecium viewed from the top. Two-foci = bilateral symmetry—one plane of symmetry; four-foci = biradial symmetry—two planes of symmetry; ring = radial symmetry—≥3 planes of symmetry; (bottom) false-coloured scanning electronic micrograph (SEM) of wild type at stage 11. Stigma (orange), style (red), valves (light blue), valve margins (green), replum (violet), including GUS-stained cross-sections of the pATHB4:GUS reporter shown for radially symmetric style (top) and bilaterally symmetric ovary (bottom). Scale bars represent 50 µm. Double-headed arrows indicate the polarity axes: A apical, B basal, M medial, L lateral, Ab abaxial, Ad adaxial. b Optical images of Toluidine blue-stained cross-sections of stage-12 style (top panels; scale bars represent 100 μm) and SEM images (middle and bottom panels) of Col-0 (left), hat3 athb4 (centre) and spt (right) at stage 9 (middle; scale bars represent 20 μm) and stage 12 (bottom; scale bars represent 100 μm). Red arrows indicate the different positions of the split style in the mutant backgrounds. c Optical images of GUS-stained gynoecia of pATHB4:GUS (top), pHAT3:GUS (middle) and pSPT:GUS (bottom) lines at stage 9 (left) and stage 12 (right) of gynoecium development. Scale bars represent 20 µm (left, stage 9) and 50 µm (right, stage 12). b , c Similar results were obtained from four independent experiments. Sections in ( a , b ) were made using samples from two of the four biological replicates in ( b , c ). d Confocal (top) and SEM (bottom) images of pAS2:HAT3:YFP/hat3 athb4 gynoecia at stage 9 (top) and stage 12 (bottom) of development. Scale bar represents 100 µm. Similar results were obtained from three independent experiments. Full size image HAT3 and ATHB4 HD-ZIP II coordinate adaxial polarity during radial symmetry establishment in the Arabidopsis gynoecium SPATULA ( SPT ) encodes a basic helix–loop–helix (bHLH)-type transcription factor required for proper gynoecium development in Arabidopsis [12] . Compared to wild-type, gynoecia from spt mutants exhibit defects in symmetry transition and the apex remains unfused [6] , [12] (Fig. 1b ). This split-style phenotype is due to the formation of a cleft in the medial region, and this defect is strongly exacerbated by combining the spt mutant with mutations in another bHLH transcription factor gene, INDEHISCENT ( IND ) [13] . The SPT/IND module functions cooperatively to mediate their activities in organ development, at least partially by affecting auxin distribution [6] , [13] , [14] . In both spt and ind spt mutants, the stepwise auxin distribution is blocked at the lateral two-foci stage, therefore failing to go through the four-foci stage and prevented from reaching the ring-formed auxin distribution required to complete the radialisation process [4] SPT has previously been proposed to function in diverse biological processes by forming interactions with process-specific bHLH proteins. Among identified SPT interactors, bHLH transcription factors belonging to the HECATE (HEC) subfamily are required for gynoecium development [15] , [16] . Interestingly, scanning electron microscopy of a hec1,2,3 triple mutant showed that growth is retarded in the lateral region, leading to a style that is diagonally split (Supplementary Fig. 1 ). Moreover, the auxin distribution in this triple mutant reaches the four-foci stage (i.e. a step further in the distribution of auxin compared to spt and spt ind mutants), but it is blocked from completing the auxin ring [16] . In addition to SPT–HEC protein interactions, SPT and HEC genes also interact genetically [16] . However, the mechanistic significance of these interactions in the bilateral-to-radial symmetry transition of the gynoecium apex is unknown. Two genes encoding HD-ZIP II family transcription factors were previously identified as direct downstream targets of both SPT and HEC proteins [17] , [18] . These two genes, HAT3 and ATHB4 , are involved in leaf abaxial/adaxial patterning [19] , [20] , shade-avoidance response [21] , auxin-regulated developmental processes [22] , [23] , and symmetry transition at the gynoecium apex as shown by the split-style phenotype of the hat3 athb4 double mutant [17] . Interestingly, we found this gynoecial split to occur diagonally with respect to the medio-lateral axis (Fig. 1b and Supplementary Fig. 2 ), suggesting that HAT3 and ATHB4 control symmetry transition in a spatial location different from SPT. The diagonal indentations in hat3 athb4 are similar to the split observed in gynoecia of the hec1/2/3 triple mutant (Supplementary Fig. 1 ), and a phenotype that also resembles loss-of-function mutants in the adaxial factors NUBBIN and JAGGED [24] . We therefore hypothesise that HAT3 and ATHB4 may have key roles downstream of the SPT/HEC module in coordinating the adaxial–abaxial axis during radial symmetry establishment, presumably via regulation of auxin dynamics. To sustain this role, we observed expression of both pHAT3:GUS ( n = 44/53) and pATHB4:GUS [22] ( n = 34/40) reporter lines in the gynoecium from early developmental stages, specifically restricted to the adaxial side of the two lateral valves (stage 9 in Fig. 1b and Supplementary Fig. 3a ). Similar to SPT expression [25] ( n = 23/23), the expression of HAT3 ( n = 45/47) and ATHB4 ( n = 48/50) was also detected in the medial tissues, including the apex of the gynoecium at later developmental stages (stage 12 in Fig. 1b and Supplementary Fig. 3a ). Moreover, by analysing the pHAT3:HAT3:YFP and pATHB4:ATHB4:GUS transgenic lines in a wild-type background, we confirmed that the distribution of HAT3 and ATHB4 protein followed by the gene expression domains (Supplementary Fig. 3b ). To corroborate the hypothesis that both factors function cell autonomously, at least partially, from the adaxial tissues, we performed tissue-specific complementation experiment whereby HAT3 was expressed under the control of the adaxial-specific ASYMMETRIC LEAVES 2 ( AS2 ) promoter [26] . Our results showed that adaxially driven expression of HAT3 is sufficient to recover cotyledon, leaf, and gynoecium defects in the hat3 athb4 background (Fig. 1d and Supplementary Fig. 4 ). This suggests that the expression of HAT3 and ATHB4 in the adaxial domain is required for radialisation of the style and to maintain an adaxial/abaxial axis during the patterning process. SPT and HEC promote HAT3 and ATHB4 expression in the style and sustain organ radialisation We then tested whether HAT3 and ATHB4 expression is regulated by SPT and HEC1,2,3 transcription factors. Quantitative reverse transcription-polymerase chain reaction (qRT-PCR) experiments on RNA extracted from inflorescences revealed a significant reduction in both HAT3 and ATHB4 transcript levels in the hec1,2,3 triple mutant (Fig. 2a ). This result was confirmed at the tissue-specific level using GUS reporter lines, which showed dramatic downregulation of HAT3 and ATHB4 expression in hec single and multiple mutant gynoecia (Fig. 2b ). While qRT-PCR experiments revealed a significant reduction in ATHB4 but not HAT3 expression in the spt mutant (Fig. 2a ), both pHAT3:GUS ( n = 39/44) and pATHB4:GUS ( n = 34/38) reporters exhibited reduced expression in spt gynoecia (Fig. 2b ). Moreover, pHAT3:GUS and pATHB4:GUS expression was undetectable in the spt hec1 double mutant ( n = 27/30) and in spt hec1,2,3 + /− ( n = 25/30), respectively (Fig. 2b ). These results are therefore in agreement with HAT3 and ATHB4 being synergistically regulated by SPT [17] and HEC1 [18] during gynoecium development. Fig. 2: SPT/HEC synergistic control of HAT3 and ATHB4 expression and genetic analyses. a qRT-PCR of HAT3 and ATHB4 in Col-0, spt and hec1,2,3 mutant inflorescences normalised against UBIQUITIN10 . The centre for the error bars represents mean, while error bars represent SD; * p < 0.05, *** p < 0.001, **** p < 0.0001, ns indicates no statistically significant difference (two-sided Student’s t test), n = 3 technical replicates. The panel displays similar results obtained from one of three biological replicates analysed, and up to six technical replicates for each gene and for each biological replicate were performed. b Optical images of stage-12 gynoecia showing pHAT3:GUS (top) and pATHB4:GUS (bottom) expression in Col-0, spt and combinations of hec1,2,3 and spt mutants, as depicted on individual panels. c SEM images of stage-12 gynoecia of Col-0, spt , spt hat3 , spt athb4 , hat3 athb4 and spt hat3 athb4 . Scale bars represent 100 µm. b , c Similar results were obtained from three independent experiments. d SEM images of stage-13 styles of ATHB4 ( XVE::ATHB4 and 35S::ATHB4:GR ) and HAT3 ( XVE::HAT3 and 35S::HAT3:GR ) overexpression lines in spt background, treated with either 20 µM β-estradiol (top) or 10 µM DEX (bottom). Scale bars represent 100 µm. e Quantification of the radial (orange bars) and split (blue bars) style phenotype of HAT3 and ATHB4 overexpression lines ( XVE::HAT3 , XVE::ATHB4 , 35S::HAT3:GR and 35S::ATHB4:GR) in spt background treated with mock, β-estradiol and DEX. Phenotypic classes were compared using contingency 2 × 2 tables followed by Pearson’s χ 2 test. Two-tailed P values are as follows: spt-12 XVE::ATHB4 β-estradiol vs spt-12 β-estradiol P < 0.00001 (§); spt-12 XVE::HAT3 β-estradiol vs spt-12 β-estradiol P < 0.00001 (#); spt-12 35S::ATHB4:GR DEX vs spt-12 DEX P < 0.00001 (*); spt-12 35S::HAT3:GR DEX vs spt-12 DEX P < 0.00001 (^). P values < 0.01 were considered as extremely statistically significant. Full size image Since a genetic interaction between SPT and the HEC genes has been reported [16] , we took a genetic approach to investigate the biological relevance of the SPT/HEC-mediated control of HAT3 and ATHB4 gene expression. We first crossed hat3 athb4 with spt and found that the triple hat3 athb4 spt mutant showed an additive effect, exhibiting both medial and diagonal clefts at their apices (Fig. 2c ). If SPT and HECs mediate at least part of their functions in gynoecium formation via their synergistic regulation of HAT3 and ATHB4 , it is possible that the ectopic expression of HAT3 and ATHB4 would rescue the gynoecium defects in spt mutant. We sought to test this by producing inducible overexpression lines of both HD-ZIP II genes. First, we found that inducing either of these two HD-ZIP II -encoding genes led to an increase in the frequency of radially symmetric styles in the spt mutant background (Fig. 2d, e and Supplementary Fig. 5 ). However, in contrast to the published effect of IND overexpression [14] , ectopic induction of HAT3 and ATHB4 was insufficient to impose radial symmetry throughout the gynoecium (Supplementary Fig. 6a ). Also, the rescue of the spt defects was not extended to the septum, which remained unfused similar to the spt control (Supplementary Fig. 5a ). Interestingly, the simultaneous overexpression of HAT3 and ATHB4 in XVE::HAT3 × XVE::ATHB4 (F 1 ) seedlings enhanced the complexity in leaves by augmenting the leaf bilateral symmetry (Supplementary Fig. 6b ), similarly to pin mutants [27] , although not affecting gynoecium development (Supplementary Fig. 6a ). Altogether, these data confirm that HAT3 and ATHB4 function downstream of the SPT/HEC module and reveal the relevance of this regulatory interaction at the gynoecium apex. 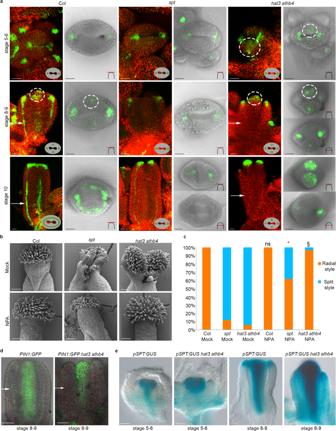Fig. 3: HAT3 and ATHB4 control auxin dynamics allowing a biradial-to-radial symmetry transition of auxin distribution. aConfocal images ofDR5rev::GFPin Col-0 (left),spt(centre) andhat3 athb4(right) at stages 5 and 6 (top), stages 8 and 9 (middle) and stage 10 (bottom) of gynoecium development. In the side view pictures (black background), chlorophyll autofluorescence is shown in red, while the gynoecium outline indicates the top-view of auxin dynamics. In the merged confocal/bright field top view pictures (light background), the schematic drawings in the bottom right corner indicate the confocal plane of the images. Dashed circles indicate the medial auxin foci. White arrows indicate the adaxial valve tissues. Scale bars represent 20 μm. Similar results were obtained from four independent experiments.bSEM images of Col-0 (left),spt(centre) andhat3 athb4(right) at stage 12 treated with mock (top) or 100 µM NPA (bottom). Scale bars represent 100 μm.cQuantification of the radial (orange bars) and split (blue bars) style phenotype of Col,sptandhat3 athb4treated with 100 µM NPA or mock. Phenotypic classes were compared using 2 × 2 contingency tables followed by Pearson’sχ2test. Two-tailedPvalues are as follows: Col NPA vs Col mock,P= 1 (ns, no statistically significant difference);spt-12NPA vsspt-12mock,P< 0.00001 (*);hat3 athb4NPA vshat3 athb4mock,P< 0.00001 (§).Pvalues < 0.01 were considered as extremely statistically significant. Similar results were obtained from three independent experiments.dPIN1:GFPexpression in wild-type (left) andhat3 athb4(right) gynoecia at stages 8 and 9 of development. White arrows indicate the adaxial valve tissues. Scale bars represent 50 μm.epSPT:GUSexpression in wild-type andhat3 athb4gynoecia at stages 5 and 6 (left) and stages 8 and 9 (right) of development. Scale bars represent 20 μm.d,eSimilar results were obtained from two independent experiments. 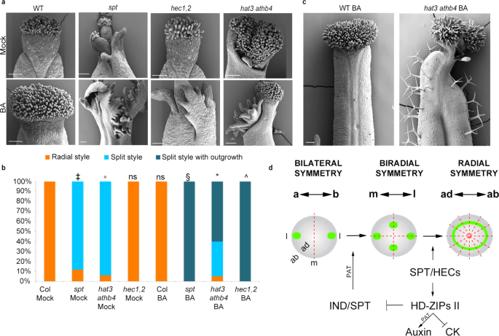Fig. 4: HAT3 and ATHB4 suppress sensitivity to cytokinin. aSEM images of stage-13 gynoecia of Col-0 wild-type,sptsingle mutant,hec1,2andhat3 athb4double mutants treated with mock (top) or 50 µM of cytokinin (BA) (bottom). Scale bars represent 100 µm.bQuantification of cytokinin (BA) effect on gynoecium apex development of genotypes depicted on the graph. Phenotypic classes were compared using 3 × 2 contingency tables followed by Pearson’sχ2test. Two-tailedPvalues are as follows:spt-12Mock vs Col Mock,P< 0.00001 (‡);hat3 athb4Mock vs Col MockP< 0.00001 (°);hec1,2Mock vs Col MockP= 1 (ns, no statistically significant difference); Col BA vs Col mock,P= 1 (ns);spt-12BA vsspt-12mock,P< 0.00001 (§);hat3 athb4BA vshat3 athb4mock,P< 0.00001 (*);hec1,2BA vshec1,2mock,P< 0.00001 (^).Pvalues < 0.01 were considered as extremely statistically significant.cSEM images of stage-13 gynoecia of wild-type (left) andhat3 athb4(right) treated with 50 µM of BA, showing the occasional trichome formation on the valves of the hypersensitive double mutant. Scale bars represent 100 μm. Similar results were obtained from two independent experiments.dModel showing the genetic regulation of consecutive transitions of auxin signalling (green) at the gynoecium apex (grey outline—top view). Double-head arrows represent the polarity axis; a apical domain, b basal domain, m medial domain, l lateral domain, ab abaxial domain, ad adaxial domain. Dashed red lines represent the planes of symmetry along the medio-lateral axis. PAT polar auxin transport, CK cytokinin. HAT3 and ATHB4 facilitate radial symmetry by controlling polar auxin transport We next investigated whether HAT3 and ATHB4 coordinate radial symmetry establishment via regulation of auxin dynamics. During wild-type gynoecium development, auxin accumulation is highly dynamic as shown by the analysis of the auxin signalling reporter DR5rev::GFP (Fig. 3a ) [6] , [10] , [11] . The spt mutant fails to accumulate auxin in the medial foci, leading to a ‘split-style’ phenotype in the medial apical part of the young gynoecium [6] (Figs. 1 b and 3a ). At early stages of hat3 athb4 development, the establishment of the two lateral foci was not affected (Fig. 3a ). These foci are important to sustain apical–basal growth, and accordingly, this mutant exhibited correct bilateral symmetry in the ovary (Supplementary Fig. 7 ). However, while the spt mutant is blocked at the two-foci stage, the hat3 athb4 mutant can advance to the four-foci stage, but fails to establish the ring-formed auxin maximum at the gynoecium apex (Fig. 3a ). Interestingly, the medial DR5rev::GFP foci are already observed at stages 5 and 6 in the hat3 athb4 mutant gynoecia ( n = 17/19 samples; Fig. 3a ), whereas they appear at stages 8 and 9 in wild type ( n = 20/24; Fig. 3a ). Fig. 3: HAT3 and ATHB4 control auxin dynamics allowing a biradial-to-radial symmetry transition of auxin distribution. a Confocal images of DR5rev::GFP in Col-0 (left), spt (centre) and hat3 athb4 (right) at stages 5 and 6 (top), stages 8 and 9 (middle) and stage 10 (bottom) of gynoecium development. In the side view pictures (black background), chlorophyll autofluorescence is shown in red, while the gynoecium outline indicates the top-view of auxin dynamics. In the merged confocal/bright field top view pictures (light background), the schematic drawings in the bottom right corner indicate the confocal plane of the images. Dashed circles indicate the medial auxin foci. White arrows indicate the adaxial valve tissues. Scale bars represent 20 μm. Similar results were obtained from four independent experiments. b SEM images of Col-0 (left), spt (centre) and hat3 athb4 (right) at stage 12 treated with mock (top) or 100 µM NPA (bottom). Scale bars represent 100 μm. c Quantification of the radial (orange bars) and split (blue bars) style phenotype of Col, spt and hat3 athb4 treated with 100 µM NPA or mock. Phenotypic classes were compared using 2 × 2 contingency tables followed by Pearson’s χ 2 test. Two-tailed P values are as follows: Col NPA vs Col mock, P = 1 (ns, no statistically significant difference); spt-12 NPA vs spt-12 mock, P < 0.00001 (*); hat3 athb4 NPA vs hat3 athb4 mock, P < 0.00001 (§). P values < 0.01 were considered as extremely statistically significant. Similar results were obtained from three independent experiments. d PIN1:GFP expression in wild-type (left) and hat3 athb4 (right) gynoecia at stages 8 and 9 of development. White arrows indicate the adaxial valve tissues. Scale bars represent 50 μm. e pSPT:GUS expression in wild-type and hat3 athb4 gynoecia at stages 5 and 6 (left) and stages 8 and 9 (right) of development. Scale bars represent 20 μm. d , e Similar results were obtained from two independent experiments. Full size image We therefore next tested whether the defect in auxin distribution is causative of the hat3 athb4 gynoecium phenotype. To this end, wild-type hat3 athb4 and spt mutants were treated with 1-naphthylphthalamic acid (NPA), an inhibitor of polar auxin transport [28] . NPA has previously been shown to inhibit auxin transport from the gynoecium base towards the apex, thereby causing developmental defects along the apical–basal axis of the gynoecium, leading to a reduction in the size of the ovary [5] (Supplementary Fig. 7 ). In contrast, the application of NPA was previously reported to rescue the split style of the spt mutant [5] as well as that of other mutants with apical defects [29] . Under our experimental conditions, 100 μM NPA spray applications were able to complement 26 of the 42 spt mutant styles analysed (61.9%) (Fig. 3b, c ). Moreover, the NPA applications rescued the split-style defects in 32 out of 33 hat3 athb4 double mutants (96.9%) (Fig. 3b, c ). In addition to the style, hat3 athb4 showed hypersensitivity to NPA application also along the apical–basal axis, as shown by the strongly decreased ovary when compared to wild type (Supplementary Fig. 7 ), suggesting that the main downstream activity of HAT3 and ATHB4 is to control auxin distribution via regulation of the polar auxin transport. This is in line with the previously identified role of HAT3 and ATHB4 as coordinators of apical embryo development via regulating the PIN1-mediated auxin accumulation [22] , [23] . Therefore, we next analysed PIN1:GFP expression in wild-type and hat3 athb4 gynoecia and confirmed a strong reduction in the number of mutant organs showing fluorescent signal specifically in the adaxial tissues of the valves. Only 9 out of 46 hat3 athb4 gynoecia analysed (19.5%) retained PIN1:GFP expression in the valves compared to 29 of the 33 wild-type gynoecia (88%) (Fig. 3d ). These data correlate with a strong reduction of DR5rev::GFP in the hat3 ahtb4 valves (Fig. 3a ), and hypersensitivity of the double mutant to NPA application (Supplementary Fig. 7 ), confirming a role for HAT3 and ATHB4 in controlling auxin distribution in the gynoecium. HAT3 and ATHB4 repress SPT expression and coordinate growth along polarity axes The presence of medial auxin foci in the hat3 athb4 double mutant correlates with proper development of the medial style, whereas lack of medial foci in the spt mutant leads to a split in this position (Fig. 1b ). Interestingly, the premature emergence of the medial foci in hat3 athb4 double mutant (Fig. 3a ) led us to hypothesise a negative feedback loop actioned by the adaxial regulators HAT3 and ATHB4 on the medial determinant, SPT, enabling growth at the medial axis of the HD-ZIPs-II double mutant apexes (Supplementary Fig. 2 ). Thus, we analysed the expression of the pSPT:GUS reporter in the hat3 athb4 mutant compared to wild type and observed a stronger expression of SPT at early developmental stages of the hat3 athb4 mutant gynoecia ( n = 25/27) (Fig. 3e ). Comparing gynoecia from the hat3 athb4 double mutant to the hat3 athb4 spt triple mutant confirms that SPT upregulation in the hat3 athb4 background contributes to the sustained radial growth in the medial–apical region of the mutant gynoecia (Fig. 2c ). Altogether, whilst demonstrating that HAT3 and ATHB4 control auxin distribution in the gynoecium apex, these data show that HAT3 and ATHB4 HD-ZIP II proteins are required to coordinate growth along the medio-lateral and adaxial–abaxial polarity axes during radialisation of the style, functioning at least partially in a cell-autonomous manner from adaxial domains (Fig. 1d ). Our results show that HAT3 and ATHB4 are key coordinators of adaxial polarity during organ symmetry establishment. Their role is sustained via precise spatio-temporal expression patterns, promoting dynamic auxin distribution and ultimately fine-tuning organ shape and function. HAT3 and ATHB4 control cytokinin sensitivity downstream of SPT/HEC SPT and HECs are key regulators of the delicate balance between auxin and cytokinin required for gynoecium patterning [16] , [30] , [31] , [32] . We therefore tested whether HAT3 and ATHB4 contribute to this function. In agreement with previous results, 100% of the hec1,2 ( n = 80) and spt ( n = 80) gynoecia showed hypersensitivity to cytokinin application [16] , leading to apically unfused organs and extensive tissue proliferation at their tip (Fig. 4a, b ). In hat3 athb4 mutant gynoecia, we observed an intermediate effect with outgrowths of split apices in the diagonal part (48 of 80 gynoecia analysed), while no changes were observed at the medial region (Fig. 4a, b ), where SPT is upregulated (Fig. 3e ). These data suggest a role for HAT3 and ATHB4 in modulating cytokinin levels downstream of SPT/HEC in a spatially specific manner. Moreover, cytokinin treatments led occasionally to trichome formation on the abaxial side of hat3 athb4 valves, which was not observed in cytokinin-treated wild-type gynoecia (Fig. 4c and Supplementary Fig. 8 ). This phenotype has been associated with cytokinin hypersensitivity [33] , [34] , [35] , and suppression of trichome fate at the abaxial epidermis of the gynoecium was shown to be controlled by the abaxial-identity factor, KANADI1, in a cytokinin-regulated fashion [33] . Taken together, these results indicate that HAT3 and ATHB4 contribute to controlling the hormonal balance between auxin and cytokinin to coordinate the body-axis formation and symmetry establishment downstream of SPT and HEC proteins (Fig. 4d ). Fig. 4: HAT3 and ATHB4 suppress sensitivity to cytokinin. a SEM images of stage-13 gynoecia of Col-0 wild-type, spt single mutant, hec1,2 and hat3 athb4 double mutants treated with mock (top) or 50 µM of cytokinin (BA) (bottom). Scale bars represent 100 µm. b Quantification of cytokinin (BA) effect on gynoecium apex development of genotypes depicted on the graph. Phenotypic classes were compared using 3 × 2 contingency tables followed by Pearson’s χ 2 test. Two-tailed P values are as follows: spt-12 Mock vs Col Mock, P < 0.00001 (‡); hat3 athb4 Mock vs Col Mock P < 0.00001 (°); hec1,2 Mock vs Col Mock P = 1 (ns, no statistically significant difference); Col BA vs Col mock, P = 1 (ns); spt-12 BA vs spt-12 mock, P < 0.00001 (§); hat3 athb4 BA vs hat3 athb4 mock, P < 0.00001 (*); hec1,2 BA vs hec1,2 mock, P < 0.00001 (^). P values < 0.01 were considered as extremely statistically significant. c SEM images of stage-13 gynoecia of wild-type (left) and hat3 athb4 (right) treated with 50 µM of BA, showing the occasional trichome formation on the valves of the hypersensitive double mutant. Scale bars represent 100 μm. Similar results were obtained from two independent experiments. d Model showing the genetic regulation of consecutive transitions of auxin signalling (green) at the gynoecium apex (grey outline—top view). Double-head arrows represent the polarity axis; a apical domain, b basal domain, m medial domain, l lateral domain, ab abaxial domain, ad adaxial domain. Dashed red lines represent the planes of symmetry along the medio-lateral axis. PAT polar auxin transport, CK cytokinin. Full size image In conclusion, our work reveals a mechanism for coordinating symmetry transition and axis polarity to complete the bilateral-to-radial transition of the Arabidopsis style. We propose a model in which SPT functions with process-specific bHLH transcription factors in two consecutive steps to control auxin distribution (Fig. 4d ). First, SPT and IND facilitate a bilateral-to-biradial transition by promoting the formation of auxin maxima in a four-foci biradial pattern [7] . Subsequently, SPT in concert with HEC proteins control the biradial-to-radial symmetry transition, thus establishing the ring-shaped auxin maximum and restricting cytokinin sensitivity (Fig. 4d ). This regulatory module also controls the expression of the adaxial regulators HAT3 and ATHB4 to coordinate the adaxial–abaxial and medio-lateral polarity axes, thereby providing a molecular framework to facilitate bilateral-to-radial symmetry transition of the style required for successful reproduction. Plant materials and growth conditions Plants were grown on soil in long-day conditions (16 h light/8 h dark) in controlled environment rooms. The following loss-of-function mutant lines spt-12 [36] (WISCDSLOX386E06), hat3 athb4 [22] (Salk_014055; Salk_104843), and hec1,2,3 [16] (GK_297B10; SM_3_17339; SALK_005294) and overexpressing XVE::HAT3 [22] line were in Col-0 background, and reporter lines of pATHB4:GUS [22] , pSPT:GUS [25] , PIN1:GFP [37] , and DR5rev::GFP [37] were employed. DNA constructs XVE::ATHB4 was constructed as follows: the complete CDS of ATHB4 (TAIR, AT2G44910) was amplified with Apa I and Spe I ends using the primers AB4-S: AATTGGGCCCATGGGGGAAAGAGATGAT and AB4-AS: GGATACTAGTCTAGCGACCTGATTTTTGCT and cloned into the XVE vector pER8 [38] in order to obtain an ER-inducible form of ATHB4. To generate the pHAT3:GUS transcriptional fusion, a DNA fragment spanning from −2094 to +3 (ATG) of HAT3 (At3G60390) was amplified using the primers HT3-BP1, GGGGACAAGTTTGTACAAAAAAGCAGGCTTCGAGCGTTGAATAAGTGTGTTAA and HT3-BP2, GGGGACCACTTTGTACAAGAAAGCTGGGTCCATTTTTCTCAACCCCAGAA, and cloned with Gateway™ technology into the pMDC163 vector [38] . The pHAT3:HAT3:YFP translational fusion was constructed as follows: first, the putative promoter of HAT3 was extended from −1768 to −5066 bp in the construct pHAT3:HAT3:GFP pMDC107 [22] . Then, an intermediate construct was generated in pBKS II plasmid by separate rounds of PCR and cloning, containing the HAT3 gene from Bst BI unique site to the stop codon (excluded), a 9x alanine linker, the EYFP CDS, and a 3 ′ UTR portion of HAT3 . Finally, the fragment HAT3:ala9:EYFP -3′ HAT3 was cut with Bst BI and Kpn I and introduced into the plasmid generated in the first step. Amplifications were performed using the primers: HAT3 Pme I for, AAGTTTAAACGATGTATTGTCCTGATGGTTC and HAT3 Pac I rev, GGTTAATTAATGATGACTCCATATATG; Spe I HAT3 3′utr fwd, AAAC*TAGTCTAAAGATAATAGGTTTGGTGATTTG (* indicates a mutation introduced in the original HAT3 sequence to generate the Spe I site) and Kpn I HAT3 3′utr rev, AAGGTACCTCCAGTTCGATTTGGTAGAAAC. The pATHB4:ATHB4:GUS translational fusion was constructed as follows: first, a DNA fragment containing the ATHB4 genomic sequence spanning from −1990 to +1635 bp was amplified from genomic DNA (Col-0) and fused to GFP in the pMDC107 vector using Gateway™ technology. Primers on the genomic DNA were as follows: −1990 ATHB4 F, CTACACTCTCTCCCACACCATTCACA and +1635 ATHB4 R, GCGACCTGATTTTTGCT. Then, a genomic fragment from −4874 to the Pac I site at −1148 of the genomic ATHB4 sequence was amplified from genomic DNA and added to the previous construct, exploiting the Pme I site in pMDC107 and Pac I site in the ATHB4 gene, thus extending the putative ATHB4 promoter up to −4874. Then, an intermediate construct was generated in pBluescript II plasmid by separate rounds of PCR and cloning: first, the ATHB4 gene from +1422 bp, including the Bbv CI site to the stop codon (excluded), was amplified from genomic DNA inserting a 9x alanine linker. Primers used were as follows: +1422 ATHB4 F, AAGAGCTCGCTGAGGGCGTTGAAGTTG and +1635 ATHB4 R, AACGCGGCCGCAGCAGCTGCCGCAGCTGCGCGACCTGATTTTTGCTGG. Second, the GUS CDS was amplified with Not I and Bam HI extremities from pBI121 plasmid and cloned in the pBluescript II intermediate downstream of the ATHB4 fragment. Third, a 3 ′ UTR portion of ATHB4 was amplified from genomic DNA and cloned downstream of the GUS CDS in the intermediate plasmid. Primers were as follows: Xcm I-GUS_TAG-3′UTR, CCCGGGCCACCGGCGGCATGGAGGGAGGCAAACAATAGGGAAGGAGTATCTTCGGT and 3′UTR-X2- Eco RI, CCCGGGGATATCCCACCATGTTGGGTTGAATTGAACATTAAGAGACTG. Finally, the fragment ATHB4:ala9:GUS-3 ′ UTR ATHB4 was cut with Bbv CI and Bst XI from the pBluescript II intermediate and introduced into the vector generated in the first step, cut with the same enzymes, thus substituting the GFP marker with the GUS marker and the 3 ′ UTR of ATHB4 . The pATHB4:ATHB4:GUS construct was stably transferred in Col-0. The 35S::HAT3:GR and 35S::ATHB4:GR were constructed as follows: the GUS gene was removed from the pBI121 vector using the Bam HI– Sst I restriction sites, replaced with the GR sequence and then amplified with Bam HI– Sst I restriction ends from the pTA7002 vector [39] . This vector was then cut with Xba I– Bam HI and used to insert either HAT3 cDNA or ATHB4 cDNA amplified with Xba I– Bam HI extremities. Primers used for HAT3 cDNA were as follows: HAT3 Xba I fwd, CGGCTCTAGAATGAGTGAAAGAGATGATGG and HAT3 Bam HI rev, AAATGGATCCATATGAGAACCAGCAGCAGG. Primers used for ATHB4 cDNA were as follows: ATHB4 Xba I fwd, CGGCTCTAGAATGGGGGAAAGAGATGATGG and ATHB4 Bam HI rev, AAATGGATCCATGCGACCTGATTTTTGCTG. The pAS2:HAT3-YFP was constructed as follows: a genomic region containing the putative AS2 promoter from −3990 to −1 was amplified with Gateway TM technology and cloned into pDONR-Zeo vector. Before the AttB2 sequence, Bam HI and Sac II sites were added. Separately, an intermediate construct was generated in pBKS II plasmid by separate rounds of PCR and cloning, containing the HAT3 cDNA, a 9x alanine linker and the EYFP CDS. The HAT3:YFP fusion was then inserted downstream of the AS2 promoter in the pDONR-Zeo plasmid using the Bam HI– Sac II sites. The pAS2:HAT3:YFP fragment was then introduced into the pMDC99 vector [40] . Primers for AS2 promoter were as follows: pAS2 fwd, TGGTAGCTAGCGTTGTTGACA and pAS2 rev, TTTAATGACTTGAAAATGGAG. All transgenic lines used were in the Col-0 background, with the exception of pAS2:HAT3:YFP , which was stably transformed in the hat3 athb4 background. The pHAT3:HAT3:YFP and the pATHB4:ATHB4:GUS constructs were able to completely rescue the hat3 athb4 mutant phenotype (70 hat3 athb4 HAT3::HAT3:YFP lines out of 70 and 50 hat3 athb4 pATHB4::ATHB4:GUS lines out of 50 showed wild type-like gynoecia). Primers for genotyping HAT3 WT: HAT3 unC: GAAACTGTACTGCTGCACAAGTG HAT3 revC: CTTCTACTCTACCTCCTCCAACTGC hat3-3 mutant: LBb1 GCGTGGACCGCTTGCTGCAACTC in combination with HAT3 unC ATHB4 WT: ATHB4 unA: GATTGGGCAGAAGCAAAAGCTGAGGGCAAG ATHB4 revA: CCCTAGCGACCTGATTTTTGCTGG athb4-1 mutant: LBb1 GCGTGGACCGCTTGCTGCAACTC in combination with ATHB4 revA HEC1 WT: HEC1 WT fwd: TAGAAGGGAGAGAATAAGCGAG HEC1 WT rev: AATGAACACAAGCCTGATAGC hec1 mutant ( GABI-KAT line 297B10 ): hec1 MUTANT fwd: ACCACAACAACACTTACCCTTTTC hec1 MUTANT rev: ATATTGACCATCATACTCATTGC HEC2 WT: HEC2 WT fwd: CTCACAAAACCTTAACTAGATGTCTGA HEC2 WT rev: ATGCTTTCTGAATCCAACACCC hec2 mutant (T-DNA SM_3_17339): hec2- MUTANT fwd: CCGACACTCTTTAATTAACTGACACTC in combination with HEC2 WT rev primer HEC3 WT: HEC3 WT fwd: TCTTTATTTTTTCTCCGAACCA HEC3 WT rev: AAGCCGTATCCATTTTAGTGCC hec3 mutant (SALK_005294 line): hec3 MUTANT fwd: GTTCACGTAGTGGGCCATC in combination with HEC3 WT rev primer SPT WT SPT WT fwd: GAAGAAGCAGAGAGTGATGGGAGA SPT WT rev: TGACTTGGAAGAGGGAGCTTCA spt-12 mutant: p745: AACGTCCGCAATGTGTTATTAAGTTGTC in combination with SPT WT fwd primer Toluidine blue staining Tissues were fixed for 16 h at 25°C in 3.7% formaldehyde, 5% acetic acid, and 50% ethanol and subsequently dehydrated through an ethanol series until 70%. The tissues were embedded in paraffin. An RM 2125 rotary microtome (Leica) was used to make 10 µm transverse sections of Col, spt-12 and hat3 athb4 gynoecia at stage 12. Paraffin was removed from the sections by two rounds of incubation in 100% Histoclear (National Diagnostics) for 10 min at room temperature, followed by two washes in 100% ethanol for 2 min at room temperature, air-dried for 30 min and stained for 10 min by an aqueous solution containing 0.005% Toluidine blue O (Acros Organics). Slides were washed for 1 min in water; sections were mounted in a histological mounting medium Histomount (National Diagnostic) and examined under Leica DM600 light microscopy. Images were taken using the Leica LAS AF7000 software. Gynoecium and seedling treatments Col-0, spt-12 and hat3-3 athb4-1 gynoecia were treated with 100 µM NPA (Duchefa Biochemie N0926), 50 or 100 µM BA (6-benzylaminoadenine, Sigma B3408) or mock, as previously described [5] , [16] . Seedlings resulting from an F1 XVE::HAT3 × XVE::ATHB4 cross were grown for 15 days on MS medium supplemented with 20 µM β-estradiol (Sigma, E8875) or mock. Inflorescences resulting from an F1 XVE::HAT3 × XVE::ATHB4 cross, as well as XVE::HAT3 /WT, XVE::HAT3 / spt , XVE:: ATHB4/WT and XVE::ATHB4 / spt inflorescences were sprayed with 20 µM β-estradiol three times every second day and gynoecia were fixed after 5 days from the last treatment. 35S::HAT3-GR / spt and 35S::ATHB4-GR / spt inflorescences were sprayed with 10 µM dexamethasone (DEX) three times every second day and gynoecia were fixed after 5 days from the last treatment. All spray treatments used 0.01% final concentration of Silwet L-77. Scanning electron microscopy Gynoecia and leaves were fixed for 16 h at 25 °C in 3.7% formaldehyde, 5% glacial acetic acid and 50% ethanol. After complete dehydration through an ethanol series until 100%, gynoecium and leaves were critical point dried. Samples were dissected and coated with gold and examined under Zeiss Supra 55VP field emission scanning electron microscope using an acceleration voltage of 3 kV. The SmartSEM software (Zeiss) was used to operate the microscope and collect the images. Gynoecia from distinct inflorescences and leaves of seedlings of several biological independent genotypes were observed and counted for their phenotype. RNA extraction and qRT-PCR Three independent biological extractions of total RNA were isolated from Col-0, hat3 athb4 and spt-12 inflorescences using RNeasy Plant Mini Kit (Qiagen), including treatment with RNase-free DNase (Qiagen) following the manufacturer’s instructions. Each RNA sample was reverse transcribed using the M-MLV Reverse Transcriptase (Promega) according to the manufacturer’s instructions. qRT-PCR experiments were performed in triplicates from each RNA sample using BRYT Green-based GoTaq qPCR Master Mix (Promega) with Chromo4 Real-Time PCR Detection System (Bio-Rad). Expression levels were calculated relative to UBIQUITIN 10 using the 2 −ΔΔct method. Primers were designed according to the recommendations of Applied Biosystems. Fifteen technical replicates for each gene were carried out using three biological replicates for each genotype. Representative results from one biological replicate are shown in the figure. Analysis was conducted using the gene-specific primers listed below: for HAT3 : HAT3 fwd, GCATCTTCATCACACATGCAG and HAT3 rev, CGATCTCATGTCCGAGTTTCT for ATHB4 : ATHB4 fwd, GCTTGAATCTTATGCCGTTGA and ATHB4 rev, TGTGCATGTGTTGAAACGAA for UBIQUITIN 10 : UB10 fwd, AGAACTCTTGCTGACTACAATATCCAG and UB10 rev, GTTAAGACGTTGACTGGGAAAACTAT GUS histochemical assay To visualise pHAT3:GUS , pATHB4:GUS , pATHB4:ATHB4:GUS and pSPT:GUS lines, GUS histochemical assay was performed using 1 mg/ml of β-glucoronidase substrate X-Gluc (5-bromo-4-chloro-3-indolyl glucuronide, Melford) dissolved in dimethyl sulfoxide. X-Gluc solution contains 100 mM sodium phosphate buffer, 10 mM EDTA, 0.5 mM K 3 Fe(CN) 6 , 3 mM K 4 Fe(CN) 6 , 0.1% Triton X-100 according to the JIC standard operating procedures. Wild-type and mutant inflorescences of pHAT3:GUS , pATHB4:GUS and pSPT:GUS were pretreated for 1 h with acetone at −20 °C, washed two times for 5 min in 100 mM sodium phosphate buffer, washed for 30 min in 100 mM sodium phosphate buffer containing 1 mM K 3 –K 4 at room temperature and then incubated between 4 and 6 h at 37 °C in the X-Gluc solution. To visualise pSPT:GUS in Col and hat3 athb4 background, samples were stained for 5 h. After staining, the samples were washed with water and then replaced with 70% ethanol until chlorophyll was completely washed out from the samples. Gynoecium was dissected, mounted in chlorohydrate (Sigma) solution and analysed using either a Leica DM6000 light microscopy (Leica LAS AF7000 software) or a Zeiss Axioscope2 Plus (ZEN 2012 software). Confocal microscopy Confocal microscopy analyses were performed on an Inverted Z.1 microscope (Zeiss, Germany) equipped with Zeiss LSM 700 spectral confocal laser scanning unit (Zeiss, Germany), using a ZEN 2012 software. GFP and EYFP samples were both excited by a 488 nm, 10 mW solid laser with emission at 492–539 nm [22] . For the lateral view of gynoecia, floral buds were dissected and mounted in water. For the top views of style region, gynoecia were dissected, mounted vertically in an agar dish and observed also using transmitting light (bright field) [6] . Statistical analysis Phenotypic classes were compared using contingency tables (either 2 × 2 or 2 × 3) followed by Pearson’s χ 2 test. Two-tailed P values < 0.0001 were considered extremely statistically significant. Statistical analysis was performed using experimental numbers obtained by counts, while graphs in figures show the percentage of the results. Figures’ panels were assembled using Photoshop®. Reporting summary Further information on research design is available in the Nature Research Reporting Summary linked to this article.